Identifying signatures of photothermal current in a double-gated semiconducting nanotube The remarkable electrical and optical properties of single-walled carbon nanotubes have allowed for engineering device prototypes showing great potential for applications such as photodectors and solar cells. However, any path towards industrial maturity requires a detailed understanding of the fundamental mechanisms governing the process of photocurrent generation. Here we present scanning photocurrent microscopy measurements on a double-gated suspended semiconducting single-walled carbon nanotube and show that both photovoltaic and photothermal mechanisms are relevant for the interpretation of the photocurrent. We find that the dominant or non-dominant character of one or the other processes depends on the doping profile, and that the magnitude of each contribution is strongly influenced by the series resistance from the band alignment with the metal contacts. These results provide new insight into the interpretation of features in scanning photocurrent microscopy and lay the foundation for the understanding of optoelectronic devices made from single-walled carbon nanotubes. A better understanding of charge transport mechanisms in nanoscale devices, especially the role of electrical contact interfaces and band bending, has been made possible in the last decade with the development of scanning photocurrent microscopy (SPCM), a dedicated local probe technique exploiting local electrical current generation from light absorption. This technique has been used for characterizing various systems such as, for example, Si nanowires [1] , [2] , [3] , colloidal quantum dots [4] , VO 2 nanobeams [5] , carbon nanotubes [6] , [7] , [8] , [9] , [10] , [11] , [12] , [13] , [14] as well as two-dimensional (2D) materials such as graphene [15] , [16] , [17] , [18] , [19] , [20] , [21] , [22] and MoS 2 (refs 23 , 24 ). In such nanoscale systems, two mechanisms have been identified for the generation of photocurrent (PC): (i) photovoltaic processes where photoexcited carriers are separated by built-in electrical fields and (ii) photothermal processes where thermoelectric forces drive carriers through light-induced thermal gradients. Single-walled carbon nanotubes (SWNTs) are long, one-dimensional conductors with a band structure ranging from quasimetallic (bandgap E g ~30 meV) to semiconducting character ( E g typically in the range of 0.1–1 eV) depending on chirality and diameter. These properties make SWNTs an ideal platform for exploring PC generation with SPCM. In early single-walled nanotubes’ SPCM work, the interpretation of PC was mostly based on photovoltaic mechanisms [6] , [7] , [8] , [9] , [11] . The importance of photothermal effects has been suggested in the context of measurements of bulk SWNT films [12] , [13] , [25] and, very recently, SPCM work on graphene and individual metallic SWNTs has emphasized the importance of photothermal mechanisms in materials with no or small bandgaps [21] , [26] . The question of the role of photothermal mechanisms in larger bandgap semiconducting nanotubes has been studied very recently in double-gated [26] and single-gated [27] suspended carbon nanotube devices. These two studies report contradictory results, leaving the understanding of fundamental mechanisms underlying PC generation in semiconducting nanotubes unclear. Here we report on the study of a suspended semiconducting nanotube device where we show that both photovoltaic and photothermal mechanisms compete in the generation of PC. In particular, we find that the dominant or non-dominant character of one or the other processes is a function of the doping profile and that the magnitude of each contribution is strongly influenced by the band alignment with the metal contacts through the resulting contact resistance. Description of the device The device consists of a suspended nanotube grown between platinum electrodes over a predefined 3-μm-wide and 1-μm-deep trench with four gates defined at the bottom (see Methods). A schematic and a scanning electron microscopy image of a typical device used in this study are shown in Fig. 1a,b , respectively. In our SPCM experiments, gate pairs G1–G2 and G3–G4 are connected to independent tunable voltage sources V G1–G2 and V G3–G4 , respectively, and source-drain voltage V SD is set to 0 V. All measurements are performed at atmospheric pressure and room temperature. A transistor characteristic curve of the device recorded by sweeping all gate voltages simultaneously with V SD =1 mV is displayed in Fig. 1c . A large conductance for holes ( R ≈300 kΩ) and a very low conductance for electrons ( R >GΩ) are observed. From the largely suppressed conductance when the device is pinched off, we conclude that the nanotube is semiconducting with a relatively large bandgap of the order of a few to several hundreds of meV [14] , consistent with the diameter distribution expected from the growth recipe used [28] . 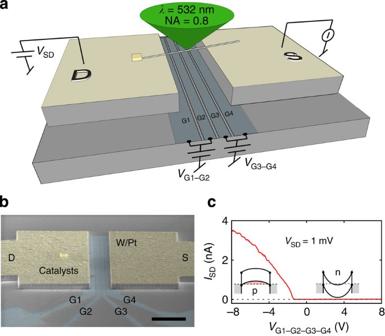Figure 1: Description and characterization of the device. (a) Schematic of the device. Gates G1–G2, G3–G4 are connected to tunable voltage sourcesVG1–G2andVG2–G3, respectively. The diffraction-limited laser spot (λ=532 nm) is accurately positioned along the suspended nanotube axis and induced photocurrent is recorded at the source (S) contact. (b) Scanning electron microscope image of a typical device. Scale bar: 5 μm. (c) Transistor curve of the device recorded by sweeping gate voltagesVG1–G2–G3–G4simultaneously withVSD=1 mV. Onsets: qualitative band diagrams in p- and n-doping regimes, corresponding to ‘ON’ and ‘OFF’ states, respectively. Figure 1: Description and characterization of the device. ( a ) Schematic of the device. Gates G1–G2, G3–G4 are connected to tunable voltage sources V G1–G2 and V G2–G3 , respectively. The diffraction-limited laser spot ( λ =532 nm) is accurately positioned along the suspended nanotube axis and induced photocurrent is recorded at the source (S) contact. ( b ) Scanning electron microscope image of a typical device. Scale bar: 5 μm. ( c ) Transistor curve of the device recorded by sweeping gate voltages V G1–G2–G3–G4 simultaneously with V SD =1 mV. Onsets: qualitative band diagrams in p- and n-doping regimes, corresponding to ‘ON’ and ‘OFF’ states, respectively. Full size image SPCM measurements PC images and corresponding qualitative band diagrams for p–n, n–n and p–p doping configurations are shown in Fig. 2 . For n–n and p–n (n–p) configurations, strong PC signatures observed at locations corresponding to local depletion regions show signs that are consistent with photovoltaic processes [7] , [14] . The PC image for the p–p configuration shows a more complex pattern with alternating sign changes along the nanotube axis. The sign of PC spots at the drain and source electrode edges is consistent with the photovoltaic mechanism. However, the sign of the PC patterns observed inside the trench cannot be explained even qualitatively by photovoltaic effects, since it indicates that electrons are travelling ‘uphill’ along the electrostatic potential profile. Similar observations have recently been reported for single-gated devices and have been attributed to photothermoelectric effects [27] . 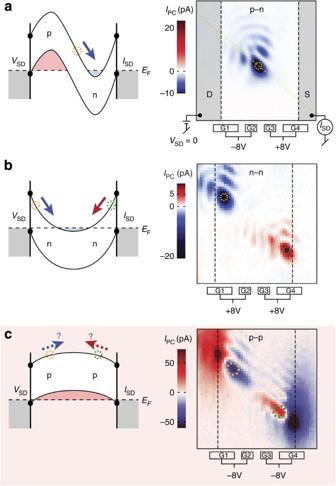Figure 2: Photocurrent images for different doping configurations. (a–c) Qualitative band diagrams (left) and photocurrent images (right) measured for p–n, n–n and p–p doping configurations, respectively. Location of trench edges (vertical black-dashed lines) and gates with applied voltages are indicated. Source (S) and drain (D) contacts with corresponding electrical connections are highlighted ina, and a yellow-dashed line shows the position of the nanotube axis. The locations of photocurrent extrema are indicated by dashed circles. The sign of the photocurrent corresponds to the conventional flow notation (red: positive, blue: negative). The arrows on the band diagrams are oriented according to the electron flow notation. Panelcillustrates the dominant photothermal mechanism observed in the p–p configuration where electrons are travelling ‘uphill’ (dashed arrows in the band diagram). Patterns around the maximum intensity PC spots in the PC images are because of diffraction effects at the trench gates14. Figure 2: Photocurrent images for different doping configurations. ( a – c ) Qualitative band diagrams (left) and photocurrent images (right) measured for p–n, n–n and p–p doping configurations, respectively. Location of trench edges (vertical black-dashed lines) and gates with applied voltages are indicated. Source (S) and drain (D) contacts with corresponding electrical connections are highlighted in a , and a yellow-dashed line shows the position of the nanotube axis. The locations of photocurrent extrema are indicated by dashed circles. The sign of the photocurrent corresponds to the conventional flow notation (red: positive, blue: negative). The arrows on the band diagrams are oriented according to the electron flow notation. Panel c illustrates the dominant photothermal mechanism observed in the p–p configuration where electrons are travelling ‘uphill’ (dashed arrows in the band diagram). Patterns around the maximum intensity PC spots in the PC images are because of diffraction effects at the trench gates [14] . Full size image In order to explore the possibility of the presence of such photothermoelectric effects in our device, we studied the PC generation mechanisms by inducing non-uniform charge-density profiles in the suspended nanotube channel using the two separate gate pairs. For this, we recorded 2D maps of the PC as a function of the gate pair voltages ( V G1–G2 and V G3–G4 ) for a fixed location of the laser spot along the nanotube axis. The resulting 2D map for the laser spot located at the centre of the suspended portion of the SWNT is shown in Fig. 3a . Four doping regions, clockwise p–n, n–n, n–p and p–p, are identified across the gate-voltage space and are delimited by two dashed black lines. A first clear feature of the image is a strongly suppressed PC in the n–n region. This can be easily understood from the very high contact resistance ( R >GΩ) measured in this regime ( Fig. 1c ). The p–n and n–p regions show PC signatures with a sign that is consistent with the photovoltaic mechanism (Note that the slight clockwise tilt angle of the strip shaped pattern arises from the fact that the laser spot is not exactly centred on the n–p (or p–n) depletion zone but is slightly shifted towards the drain contact). However, the p–p region shows PC features that are not consistent with a purely photovoltaic mechanism. This can be verified if one considers the line trace in Fig. 3b corresponding to a transition from p–n to p–p + doping configuration along the vertical dashed line in the PC map, which reveals two sign reversals of the PC signal. From a purely photovoltaic mechanism, one would expect a monotonic increase of the PC signal from the p–n minimum to a positive value in the p–p + region with a zero crossing at the symmetric p–p doping profile. This would show only one single PC sign reversal corresponding to a sign reversal of the electric field at the laser spot location. The exact same analysis applies for the PC signal recorded along the horizontal dashed line in the 2D map ( Fig. 3c ). 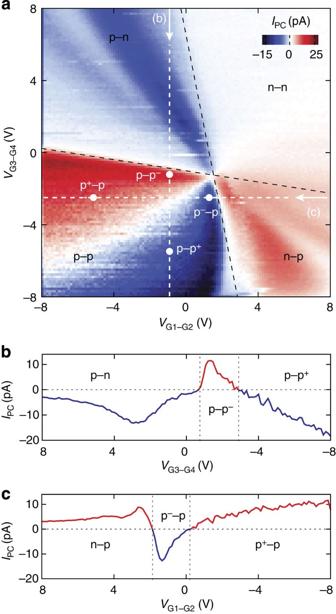Figure 3: Gate dependence of the photocurrent demonstrating a clear dominating photothermal response. (a) A 2D map of the measured photocurrent (IPC) versusVG1–G2andVG3–G4recorded with laser focussed near the middle section of the suspended nanotube, close to the p–n photocurrent minimum shown inFig. 2a. Black-dashed lines delimit four p–n, n–n, n–p and p–p doping regions. (b,c)IPCline traces recorded along the vertical, respectively, horizontal white dashed lines ina. Doping configurations of the different gate voltages are indicated by the labels inb,c. Figure 3: Gate dependence of the photocurrent demonstrating a clear dominating photothermal response. ( a ) A 2D map of the measured photocurrent ( I PC ) versus V G1–G2 and V G3–G4 recorded with laser focussed near the middle section of the suspended nanotube, close to the p–n photocurrent minimum shown in Fig. 2a . Black-dashed lines delimit four p–n, n–n, n–p and p–p doping regions. ( b , c ) I PC line traces recorded along the vertical, respectively, horizontal white dashed lines in a . Doping configurations of the different gate voltages are indicated by the labels in b , c . Full size image Model for photothermal currents From the above analysis, it is clear that the PC in the p–p region of Fig. 3 cannot be described by a photovoltaic mechanism, even at a qualitative level. In Fig. 4 , we show how the observations in Fig. 3 can be explained with a simple model where the suspended nanotube is separated in two regions of different carrier densities on the left and right sides of the laser spot. The model also includes the effect of laser heating at the junction between the two regions. The left (drain contact) and right (source contact) portions have average Seebeck coefficients S 1 and S 2 , respectively. The laser light induces a temperature increase Δ T with respect to the contacts that can be regarded as heat sinks. We consider linear temperature profiles from the S 1 – S 2 interface to the contacts [12] , [27] . Photothermal currents are induced by the local electromotive field E PT =− S ∇ T , where ∇ T is the temperature gradient along the nanotube axis and S is the Seebeck coefficient. Thus, the generated photothermal current can be expressed by I PT =− R −1 ·∫ S ( x ) ∇ T d x , where R is the overall contact resistance. 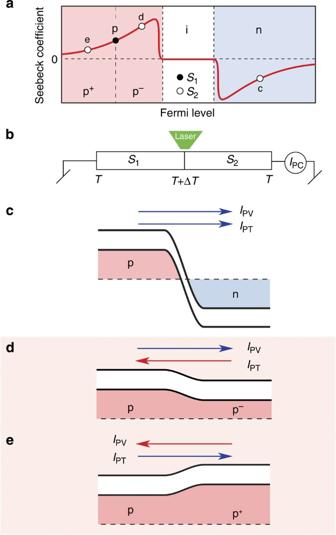Figure 4: A simple model for photothermal currents travelling against an electric field. (a) Qualitative behaviour of the Seebeck coefficient of a semiconducting carbon nanotube versus Fermi level. (b) Thermocouple model with two separately gated nanotube regions with corresponding Seebeck coefficientsS1andS2. Laser excitation region located at the two regions interface gives rise to a temperature increase ΔT. (c–e) Band diagrams for p–n, p–p−and p–p+doping configurations with corresponding photovoltaic and photothermal current arrows oriented with respect to the electronic flow notation. The colour corresponds to the current sign with respect to the conventional flow notation. Applied to our thermocouple model, we find: Figure 4: A simple model for photothermal currents travelling against an electric field. ( a ) Qualitative behaviour of the Seebeck coefficient of a semiconducting carbon nanotube versus Fermi level. ( b ) Thermocouple model with two separately gated nanotube regions with corresponding Seebeck coefficients S 1 and S 2 . Laser excitation region located at the two regions interface gives rise to a temperature increase Δ T . ( c – e ) Band diagrams for p–n, p–p − and p–p + doping configurations with corresponding photovoltaic and photothermal current arrows oriented with respect to the electronic flow notation. The colour corresponds to the current sign with respect to the conventional flow notation. Full size image The sign of the above expression (conventional flow notation) is then given by the Seebeck coefficients, whose absolute values and signs depend on the doping levels. A qualitative profile of the Seebeck coefficient as a function of the Fermi level for a semiconducting SWNT is shown in Fig. 4a [27] , [29] . Analysis and interpretation of the experimental results Band diagrams corresponding to doping configurations along the vertical line in Fig. 3a , that is, p–n, p–p − and p–p + , are drawn in Fig. 4c–e , respectively. The photothermal and photovoltaic currents are indicated with arrows oriented with respect to the electronic flow notation (colours correspond to the current sign with respect to the conventional flow notation, that is, red for positive and blue for negative). From this, we find that the photovoltaic and photothermal currents in the case of the p–n (and n–p) configuration flow in the same direction. However, we find that photovoltaic and photothermal currents are flowing in opposite directions for p–p − and p–p + (p − –p and p + –p). To understand these opposite flowing currents, it is important to contrast the mechanisms driving the two. For photovoltaic currents, electron flow is driven by differences in electrostatic voltage: electrons move to the point of lowest energy. For photothermal currents, electrons are driven by differences in chemical potential and in some cases can cause electrons to flow ‘uphill’. The photothermal current signs given by our model for gate-voltage configurations corresponding to a p-doped nanotube channel ( Fig. 4d,e ) are consistent with the experimental results (p–p region in Fig. 3a ), indicating that photothermoelectric effects are dominant in our device in this regime. From equation 1 and the maximum PC in the p–p region of ~20 pA corresponding to a Seebeck coefficient difference S 2 − S 1 ≈140 μV K −1 (ref. 29 ), we estimate the laser-induced temperature increase Δ T to be in the order of ~50 mK. This is smaller than what was reported in a previous work [26] . This could be a result of the approximation of an abrupt junction in our model, from different net laser powers reaching the sample, or from a different ratio between excitation energy and optical resonances of the nanotube. From data in Fig. 3 , it is also quite clear that the largest PC occurs in the p–p region, suggesting that photothermal mechanisms are the most dominant in our device for all gate voltages. However, we note that one has to be careful in comparing PC levels from different doping configurations of the device, since the PC is also sensitive to series resistances to the contacts. A more relevant comparison figure for different doping levels is the photo-induced voltage: for our device, in the p–n configuration, the photovoltage should be quite large, on the order of the bandgap (~100 meV). In contrast, in the p–p regions where the PC is the largest, the photothermal voltage estimated from the device resistance ( R ~300 kΩ) and observed current is on the order of ≈10 μ eV. Although the photovoltage in the p–n and n–p regions should be significantly larger than in the p–p region, the PC is comparable or smaller because of the very large n-type contact series resistance ( R >GΩ). In previous studies with graphene [21] , [30] and metallic nanotubes [26] , 2D gate maps such as the one in Fig. 3a showed a very characteristic sixfold rotational symmetry pattern that was used as a fingerprint for identifying a dominating photothermal effect. In contrast, our semiconducting suspended nanotube shows instead a more fourfold-like pattern. This lack of symmetry finds its origin in the fact that we are working with a semiconducting material with asymmetric n- and p-type contact resistances. In particular, the suppressed PC signal in the n–n region is because of the very large n-type contact resistance ( R > G Ω). For graphene (a semi-metal) and metallic SWNTs, the lack of an energy bandgap allows for similarly low p-type and n-type contact resistances, resulting in equal intensity PC signatures both in p–p and n–n regions of the 2D maps, thus forming a sixfold pattern. Furthermore, we note that our conclusion for dominant photothermal PC in the p-type regime is in contradiction with a recent work [26] , in which it was suggested that the photovoltaic mechanism dominates PC generation in suspended semiconducting nanotubes for all doping configurations. We address these apparent contradictory results by noting that compared with our device, the devices in ref. 26 had a much lower contact resistance for n-type doping (~100 MΩ) and a much higher resistance for p-type doping (~10 MΩ). This suggests a more symmetric effective work function alignment in their devices, with the Fermi level of the leads pinned near the mid-gap level (this difference in work function alignment is likely because of the vacuum environment and the vacuum thermal annealing procedure reported, which likely removed an adsorbed water layer on the surface of the silicon oxide in the trench). With the larger Schottky barriers for p-type doping in ref. 26 , the photothermal currents are likely suppressed to a level close to or below the noise floor of the measurement by the large series resistance to the contacts. In summary, we have shown that for the interest of interpreting the origin of PC features in SPCM with semiconducting nanotubes, photothermal effects can absolutely not be a priori excluded. Similar to systems such as graphene and metallic SWNTs, suspended semiconducting SWNTs can show strong photothermoelectric effects through the measurement of photothermal currents induced by inhomogeneous doping profiles along thermal gradients. However, the dominant or non-dominant character of photothermal currents compared with photovoltaic currents strongly depends on the doping profile of the device and on the n- and p-type contact resistances. Sample fabrication The fabrication of our device began with a p++ silicon wafer used as a backgate covered by 285 nm of thermal silicon oxide. On top of this, gate electrodes made of 5/25 nm W/Pt were defined using electron-beam lithography, followed by the deposition of a 1,100-nm-thick SiO 2 layer. A 1,000-nm-deep trench was dry-etched, leaving a thin oxide layer on top of the gates. A 5/25-nm-W/Pt layer was then deposited to serve as source and drain contacts, and a SWNT was grown at the last fabrication step at a temperature of 900 °C from patterned Mo/Fe catalysts [28] , [31] . SPCM set-up Our SPCM set-up [14] consists of a confocal microscope system with the objective (NA=0.8) illuminated by λ =532 nm continuous wave-collimated laser light. The diffraction-limited spot with a measured diameter of ~330 nm is scanned across the sample surface by means of two orthogonal galvo-mirrors ( x , y ) combined to a telecentric lens system, while the PC signal as well as the reflected light intensity are recorded simultaneously in order to determine the absolute position of the detected PC features. Measurements All measurements presented in this work are performed at atmospheric pressure and room temperature. For SPCM measurement, the source-drain voltage is maintained to 0 V and typical light intensities of 5 kW cm −2 are used. How to cite this article: Buchs, G. et al. Identifying signatures of photothermal current in a double-gated semiconducting nanotube. Nat. Commun. 5:4987 doi: 10.1038/ncomms5987 (2014).